Magnetization amplified by structural disorder within nanometre-scale interface region Direct magnetization measurements from narrow, complex-shaped antiphase boundaries (APBs; that is, planar defect produced in any ordered crystals) are vitally important for advances in materials science and engineering. However, in-depth examination of APBs has been hampered by the lack of experimental tools. Here, based on electron microscopy observations, we report the unusual relationship between APBs and ferromagnetic spin order in Fe 70 Al 30 . Thermally induced APBs show a finite width (2–3 nm), within which significant atomic disordering occurs. Electron holography studies revealed an unexpectedly large magnetic flux density at the APBs, amplified by approximately 60% (at 293 K) compared with the matrix value. At elevated temperatures, the specimens showed a peculiar spin texture wherein the ferromagnetic phase was confined within the APB region. These observations demonstrate ferromagnetism stabilized by structural disorder within APBs, which is in direct contrast to the traditional understanding. The results accordingly provide rich conceptual insights for engineering APB-induced phenomena. Understanding spin order in interface regions is vitally important for materials science and relevant technologies [1] , [2] , [3] , [4] , [5] , [6] . Considering various non-artificial interfaces, which are inevitably produced during heat treatment of specimens, the antiphase boundary (APB) has been the subject of intensive research. Of particular importance is an understanding of the relationship between the magnetism and structural disorder within APBs. For many alloys and compounds, atomic disordering in the APB region has been believed to deteriorate the ferromagnetic spin order [7] , [8] , [9] , [10] . For engineering using APBs, this relationship induces functionalities such as magnetoresistance [11] , [12] , large critical fields for magnetic saturation [13] and domain-wall pinning [14] . However, magnetic degradation in APBs may be deleterious for spintronic applications; for example, structural disorder depresses spin polarization in Heusler-type ordered alloys [15] . Thus, a challenge in materials science and technology is to explore a distinct type of APB in which the ferromagnetic spin order is not appreciably depressed; instead, the magnetization can be increased in the APB regions. In this article, we demonstrate that the magnetization is amplified by atomic disorder in the narrow APB regions produced in Fe 70 Al 30 alloy. Fe–Al alloys have been extensively studied for decades due to the extraordinary phenomena and functionalities that they demonstrate [16] , [17] , [18] , [19] , [20] , [21] , [22] , [23] , [24] , [25] . These alloys are potential candidates to replace stainless steels because of properties such as their high strength, excellent corrosion resistance and low density [20] . Fe–Al alloys with specific compositions exhibit an unexpectedly high recoverable strain (~5%) due to the expansion/shrinkage of deformation-induced APBs [25] . An intriguing aspect of this alloy system is the relationship between magnetism and structural disorder, which continues to attract significant attention from researchers [16] , [17] , [18] , [19] , [20] , [22] , [23] , [24] . We can compare the B2-type ordered phase with the A2-type disordered phase in Fe 70 Al 30 alloys, as illustrated in Fig. 1a . Theory predicts significant enhancement of magnetic moment in the A2-type disordered phase [17] , [20] , [22] . Conceptually, this magnetic enhancement is due to the increased probability of achieving first-nearest Fe–Fe pairs (responsible for ferromagnetic spin order) within the crystal. It appears that the structural disorder is also relevant to the spin density wave [19] and/or spin glass-like state [18] observed in Fe–Al alloys at low temperatures. The disordered configuration can be obtained at ambient temperature either by quenching the high-temperature A2 phase or by introducing lattice imperfections (including deformation-induced APBs) by severe plastic deformation of the B2 phase [18] , [24] . 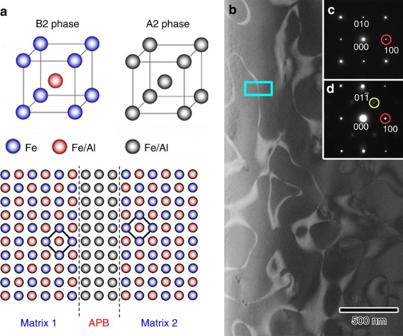Figure 1: APBs observed in the B2-type ordered Fe70Al30alloy. (a) Schematic illustrations of B2-type ordered phase, A2-type disordered phase and APB separating the left B2-type ordered region (matrix 1) from the right B2-type ordered region (matrix 2). The APBs produced by the heat treatment show a finite width, on the order of nanometres. (b) TEM image (bright-field image) revealing the locations of APBs. The image was obtained with the electron incidence slightly deviated from the [001] axis, that is, tilting the specimen made the superlattice reflections due to B2-type ordering (for example,100reflection) strongly excited. The image contrast is complementary to that of the dark-field image obtained using the superlattice reflection100. (c) Electron diffraction pattern observed in the electron incidence [001]. Superlattice reflection indicated by the red circle is due to B2-type ordering. (d) Electron diffraction pattern observed in the electron incidence [011]. Superlattice reflection indicated by the red circle is due to B2-type ordering. Weak spot indicated by the yellow circle is due to D03-type short range order. Figure 1: APBs observed in the B2-type ordered Fe 70 Al 30 alloy. ( a ) Schematic illustrations of B2-type ordered phase, A2-type disordered phase and APB separating the left B2-type ordered region (matrix 1) from the right B2-type ordered region (matrix 2). The APBs produced by the heat treatment show a finite width, on the order of nanometres. ( b ) TEM image (bright-field image) revealing the locations of APBs. The image was obtained with the electron incidence slightly deviated from the [001] axis, that is, tilting the specimen made the superlattice reflections due to B2-type ordering (for example, 100 reflection) strongly excited. The image contrast is complementary to that of the dark-field image obtained using the superlattice reflection 100 . ( c ) Electron diffraction pattern observed in the electron incidence [001]. Superlattice reflection indicated by the red circle is due to B2-type ordering. ( d ) Electron diffraction pattern observed in the electron incidence [011]. Superlattice reflection indicated by the red circle is due to B2-type ordering. Weak spot indicated by the yellow circle is due to D0 3 -type short range order. Full size image The other important source for structural disorder is thermally induced APBs, which are produced by heat treatment (via nucleation, growth and impingement of individual B2-ordered regions). As schematically shown in Fig. 1a , the thermal APB separates ordered matrix regions showing a definite change in the atomic sequence. Different from the deformation-induced APBs produced by dislocation movement, thermal APBs are believed to have a finite thickness within which the degree of atomic order is depressed [9] , [26] , [27] . In Fe–Al alloys, we accordingly expect that ferromagnetic spin order can be developed by atomic disorder within thermal APBs. This relationship, that is, ferromagnetism stabilized by thermal APBs, is unusual when compared with observations in other alloys in which the APB regions in principle deteriorate the ferromagnetic spin order [7] , [8] , [9] , [10] . Intensive studies of Fe–Al alloys are thus anticipated to provide renewed insights for materials engineering using thermal APBs. In practice, detailed examinations of APBs have been hampered by a lack of experimental tools suitable for complex-shaped, narrow interface regions. In this work, to reveal magnetism in thermal APBs in Fe 70 Al 30 , we employed techniques using advanced transmission electron microscopy (TEM), including split-illumination electron holography [28] , that enabled precise magnetic flux mapping. Structural disorder in APB region We first describe the structure of a thermal APB produced in the B2 phase. A conventional TEM image (bright-field image) determines the locations of thermal APBs, seen as bright bands in Fig. 1b . The image contrast is complementary to that of dark-field images obtained using the superlattice reflection 100 . Since this image is a projection, the APB contrast is widened when the plane is tilted away from the incident electrons. In what follows, we focus on particular APB planes that are almost parallel to the incident electrons, that is, in the edge-on condition. 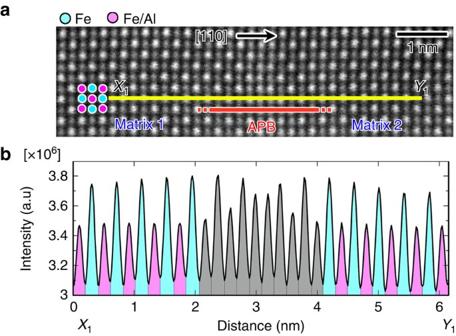Figure 2: Structure of APB produced by heat treatment in the Fe70Al30alloy. (a) Atomic-column imaging by high-angle annular dark-field scanning TEM (HAADF-STEM) with electron incidence [001]. (b) Intensity profile observed for theX1–Y1line shown ina, which traces the atomic columns of Fe (blue) and Fe/Al (pink). Difference in the peak intensity is obscured in the APB region because of atomic disordering. The image was subjected to a filtering process, in which apertures were located in all the spot positions observed in the digital diffractogram, to reduce statistical noise. Figure 2a shows atomic-column imaging by high-angle annular dark-field scanning TEM acquired from a region that includes an edge-on APB. The image intensity is approximately proportional to the square of the (averaged) atomic number in individual columns [29] . Figure 2b shows the intensity profile along the X 1 – Y 1 line crossing the APB. Both matrix regions show a well-defined B2-type superstructure made of Fe columns (blue) and Fe/Al columns (pink). In contrast, the difference in peak intensity is obscured in the APB region (grey), indicating atomic disordering (A2-type disordering) that occurs over this area. These observations can be rationalized based on the framework of classical thermodynamic theories. As indicated by Allen and Cahn [26] , a gradual change in an order parameter (as opposed to a discrete change) can reduce the free energy in the interface region. For the Fe 70 Al 30 alloy, a representative order parameter is the degree of B2-type atomic ordering. Eventually, the system favours a finite width of the APB across which atomic disordering occurs. The width of the APB, represented by grey in Fig. 2b , is ~2 nm. However, because of a gradual change in the peak intensity that may occur in the Fe/Al sites of matrix regions (in the neighbourhood of the grey peaks), it is difficult to accurately determine the terminal position of the APB. The results appear to contain an uncertainty of ~1 nm, due to the ambiguity in determining the terminal position. Considering this uncertainty, the value of the APB width is taken to be 2–3 nm in this paper. Figure 2: Structure of APB produced by heat treatment in the Fe 70 Al 30 alloy. ( a ) Atomic-column imaging by high-angle annular dark-field scanning TEM (HAADF-STEM) with electron incidence [001]. ( b ) Intensity profile observed for the X 1 – Y 1 line shown in a , which traces the atomic columns of Fe (blue) and Fe/Al (pink). Difference in the peak intensity is obscured in the APB region because of atomic disordering. The image was subjected to a filtering process, in which apertures were located in all the spot positions observed in the digital diffractogram, to reduce statistical noise. Full size image Electron energy-loss spectroscopy (EELS) was used to obtain additional information on the chemical composition within a thermal APB. 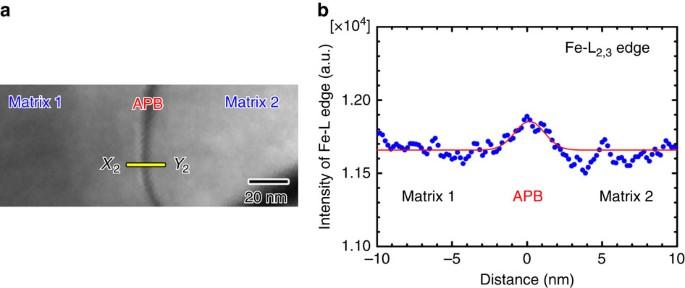Figure 3: Change in the Fe content in the APB region. (a) Conventional dark-field image showing thermal APB. (b) Plot of the intensity of the Fe-L2,3edge, observed in the EELS measurement along theX2–Y2line shown ina. The blue dots indicate observations. The red curve represents fitting using a Gaussian function. Figure 3b plots the intensity of the Fe-L 2,3 edge measured along the X 2 – Y 2 line shown in Fig. 3a . It appears that the intensity is maximized at the APB location, although the signal from EELS is noisy. Assuming that the intensity is proportional to the number of Fe atoms at individual measurement points (blue dots), the fitting curve (red line) indicates only a slight enrichment of Fe content by ~2% in the APB region, compared with the average value of the matrix. Interestingly, this result is consistent with phase-field calculations; a plausible driving force for this phenomenon is the reduction in the free-energy penalty due to the collapse of the long-range (B2-type) structural order in an APB [21] . Thus, the structure of a thermal APB in the Fe 70 Al 30 alloy can be represented in terms of three points: (1) finite width, (2) structural disorder representing the A2-type configuration and (3) slight enrichment of Fe content. Figure 3: Change in the Fe content in the APB region. ( a ) Conventional dark-field image showing thermal APB. ( b ) Plot of the intensity of the Fe-L 2,3 edge, observed in the EELS measurement along the X 2 – Y 2 line shown in a . The blue dots indicate observations. The red curve represents fitting using a Gaussian function. Full size image Ferromagnetic order stabilized in APB region The impact of a thermal APB on ferromagnetic spin order is critical. We acquired Lorentz microscopy images for a wide temperature range, from 293 to 703 K; see Fig. 4a–e . The view field is identical to that of the TEM image in Fig. 1b . Heating the specimen to 573 K intensified the stripes (the meandering bright and dark lines), which originate from deflection of incident electrons due to the Lorentz force [8] , [9] , [30] , [31] . Importantly, these striations are present in the APB locations. The observations clearly indicate the magnetic anomaly that occurs in the APB region. Further heating reduced the magnetic contrast, as demonstrated in Fig. 4d,e , due to the elimination of spontaneous magnetization in this specimen. In fact, the magnetic contrast is almost invisible in Fig. 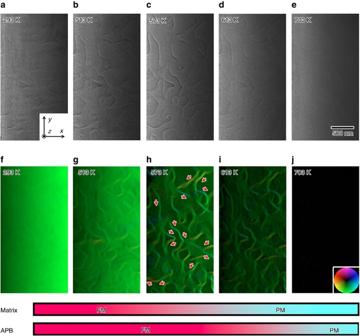Figure 4: Direct imaging of magnetization distribution in the APB region. (a–e) Lorentz microscopy images observed at 293, 513, 573, 613 and 703 K, respectively. Magnetic contrast (paired bright and dark lines) indicating the variation in local magnetic flux density can be observed along the APBs: see images ina–d. The view field is identical to that shown inFig. 1b. (f–j) Mapping of the phase gradient revealed by electron holography. The results were collected from the same area as that shown ina–e, at 293, 513, 573, 613 and 703 K, respectively. The phase gradient provides a measure of the in-plane magnetic flux density, whose direction and magnitude are represented based on the colour wheel shown inj. Undesired contribution from the mean inner potential was removed by using a reference hologram that was acquired in the paramagnetic phase at 713 K (not shown here). Undesired diffraction contrast was removed by tilting the specimen when the electron holograms were collected. FM and PM represent ferromagnetic and paramagnetic, respectively. 4e , which only shows a faint (non-magnetic) spotty pattern due to contamination that appears to form around 700 K. The absence of magnetic signals at 703 K is consistent with magnetization measurements using bulk specimens [23] , [32] ; that is, phase transition to the paramagnetic state is completed on heating the specimen to ~700 K. Figure 4: Direct imaging of magnetization distribution in the APB region. ( a – e ) Lorentz microscopy images observed at 293, 513, 573, 613 and 703 K, respectively. Magnetic contrast (paired bright and dark lines) indicating the variation in local magnetic flux density can be observed along the APBs: see images in a – d . The view field is identical to that shown in Fig. 1b . ( f – j ) Mapping of the phase gradient revealed by electron holography. The results were collected from the same area as that shown in a – e , at 293, 513, 573, 613 and 703 K, respectively. The phase gradient provides a measure of the in-plane magnetic flux density, whose direction and magnitude are represented based on the colour wheel shown in j . Undesired contribution from the mean inner potential was removed by using a reference hologram that was acquired in the paramagnetic phase at 713 K (not shown here). Undesired diffraction contrast was removed by tilting the specimen when the electron holograms were collected. FM and PM represent ferromagnetic and paramagnetic, respectively. Full size image A question thus arises as to whether the magnetization increases or decreases in the APB regions in the Fe 70 Al 30 alloys. Electron holography provides crucial information; it determines the phase shift ? of an electron that has traversed a thin-foil specimen. With reference to the x–y–z coordinate system shown in Fig. 4a (that is, x and y are parallel to the foil plane and z is along the direction of the incident electrons), ? measured in the x direction can be expressed as [30] , where C E , V 0 , t , e , ħ and B y represent a constant, the mean inner potential in the crystal, the specimen thickness, the elementary charge, Planck’s constant divided by 2 π and the y component of the magnetic flux density, respectively. The integral is carried out over the area enclosed by the paths of electrons [30] . Because of the cubic symmetry (that is, low magnetic anisotropy) in the crystal, it can be assumed that the stray magnetic field, which exits above and below the thin-foil specimen, is small compared with the significant magnetic flux density within the Fe-based alloy. Thus, B y (x) approximates the in-plane magnetic flux density, which may be varied in the APB region. To extract information on B y , we removed the undesired signal due to the electrostatic potential (that is, first term of equation (1)) by using a reference hologram acquired in the non-magnetic phase at 713 K (ref. 31 ). This process leads to a simple relationship between the phase gradient and B y multiplied by t (ref. 30 ), The value of t ( x ) was determined by cross-sectional TEM observations using the thin-foil specimen: see Supplementary Note 1 . (Once V 0 was determined by cross-sectional observations, the thickness could also be determined by using the first term of equation (1).) Similarly, ? measured in the y direction can be related to the x component of the magnetic flux density B x , Note that a minus sign in the right side of equation (3) is absent for a vector of magnetic flux ( B ), which is represented in the x–y–z coordinate system shown in Fig. 4a . Both equations (2) and (3) are consistent with the sense of the phase shift that can be observed in x and y directions, respectively. Figure 4f–j present two-dimensional mapping of the phase gradient, observed as a function of temperature. The view field is identical to that shown in Fig. 4a–e . The direction and magnitude of the phase gradient are represented based on the colour wheel shown in Fig. 4j . As seen in Fig. 4f , this area appears to be magnetized approximately in one direction indicated in green. The anomaly in the APB is not clear yet because of the significant magnetization in both the matrix and APB regions at 293 K. Significant heating reduces the magnetization in the matrix, as demonstrated by the increasing dark area in Fig. 4g–i . A noteworthy point is that magnetization in the APB remains pronounced (compared with the matrix region) at elevated temperatures, as shown in Fig. 4h,i . The results definitively indicate that ferromagnetic spin order is stabilized by the APBs. In addition, Fig. 4h,i offer essential information for developing an understanding of the ferromagnetic phase confined in the narrow, complex-shaped boundary region. In the presence of low magnetocrystalline anisotropy in the cubic system, the magnetic dipolar interaction dominates the spin alignment in the APB. The magnetization vectors accordingly trace the highly meandering APB; refer to the positions labelled with red arrows indicating local magnetic flux directions ( Fig. 4h ). As a result, the specimen shows a network of thin-layered ferromagnetic regions. Further heating makes the whole area of the specimen paramagnetic, as shown in Fig. 4j . It is likely to be that the effective Curie temperature in the APB is higher than that of the matrix by at least 30 K. The locations of APBs remain unchanged on heating to 703 K. The spatial resolution of electron holography needs to be mentioned. The resolution can be approximated as three times the fringe pitch in an electron hologram, which is produced by interference between the reference wave and the object wave [30] . The fringe pitch was 17 nm for the results shown in Fig. 4f–j . This value of the fringe pitch, which is larger than the APB width, was needed for image acquisition from a wide field of view, shown in Fig. 4 . Because of this experimental condition, the observed APB regions are broadened in Fig. 4f–i . Nevertheless, the observations clearly show the ferromagnetic phase that persists in the locations of APBs at elevated temperatures: see Fig. 4h,i . This is because the electron holography study accurately determined the phase shift in the matrix regions, the size of which (on the order of 100 nm) is sufficiently larger than the resolution. As we will demonstrate in Fig. 5a–c , the magnetic anomaly in the APB region can be recognized by the deviation of the base lines (that is, plots of the phase shift) determined for the neighbouring matrix regions. Results of high-resolution measurements shown in Fig. 5a–c will be discussed later. 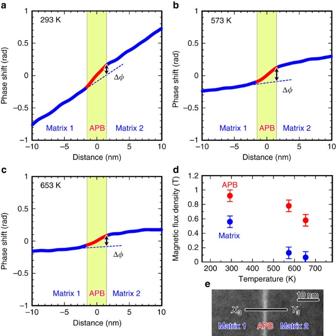Figure 5: Determination of magnetic flux density in the APB region. (a–c) Plots of the phase shift which was measured along theX3–Y3line (shown ine) at 293, 573 and 653 K, respectively. The results were acquired from the same specimen used inFigs 1and4. Blue and red curves show the matrix and APB regions, respectively. Δ? is the phase difference (between the observation and fitting curve for matrix 1 (dotted line)) observed at the terminal of the APB region. (d) Temperature dependence of the magnetic flux density determined for the APB (red) and matrix (blue). The error bars (±0.08 T) are mainly due to the uncertainty in measuring specimen thickness. (e) TEM image (bright-field image) revealing the location of the APB. The view field is identical to that indicated by the rectangle inFig. 1b. Figure 5: Determination of magnetic flux density in the APB region. ( a – c ) Plots of the phase shift which was measured along the X 3 – Y 3 line (shown in e ) at 293, 573 and 653 K, respectively. The results were acquired from the same specimen used in Figs 1 and 4 . Blue and red curves show the matrix and APB regions, respectively. Δ? is the phase difference (between the observation and fitting curve for matrix 1 (dotted line)) observed at the terminal of the APB region. ( d ) Temperature dependence of the magnetic flux density determined for the APB (red) and matrix (blue). The error bars (±0.08 T) are mainly due to the uncertainty in measuring specimen thickness. ( e ) TEM image (bright-field image) revealing the location of the APB. The view field is identical to that indicated by the rectangle in Fig. 1b . Full size image Determination of magnetic flux density in APB A big challenge in electron microscopy is to determine the magnetic flux density in the thin APB region. We plotted the phase shift ? measured along the X 3 – Y 3 line crossing the APB shown in Fig. 5e . The view field is identical to that indicated by the rectangle in Fig. 1b . Unwanted diffraction contrast was removed by tilting the specimen when the electron holograms were collected. The fringe pitch of the electron holograms was 0.8 nm (that is, resolution of 2.4 nm) when the results of Fig. 5a–c were collected. As shown for the observation at 293 K ( Fig. 5a ), the slope of ? becomes steep at the APB location. Equation (2) evaluates the magnetic flux density ( B y ) for the matrix region at 0.56 T (average for matrix 1 and matrix 2, at 293 K), which is not largely deviated from the value deduced from bulk magnetization measurements at ~0.5 T (ref. 16 ). Considering the phase difference Δ?, which represents the deviation between the observation at the APB terminal and the extrapolation for matrix 1 (that is, blue dotted line), B y for the APB was determined to be 0.92 T. Surprisingly, the magnetic flux density in the APB region is amplified by a factor of 1.6, as compared with the value for the matrix. Apinaniz et al. [22] reported a large magnetic moment of the A2-disordered phase using calculations, which was amplified by a factor of 1.9 compared with the B2-ordered phase in Fe 75 Al 25 alloys. It is likely to be that the observed B y amplification (~1.6 for Fe 70 Al 30 alloys) is not unreasonable if we assume incomplete atomic disordering in the APB region and/or imperfect ordering in the matrix area; the degree of atomic order remains to be determined in future study. It is to be noted that the specimens of Fe 70 Al 30 definitively showed B2-type ordering, as demonstrated by the sharp superlattice reflections indicated by red circles in the electron diffraction patterns ( Fig. 1c,d ). The weak spot indicated by the yellow circle in Fig. 1d implies short-range D0 3 -type ordering, which is characterized by atomic ordering within the body-centred sites [20] , [21] , [22] , [23] . Following calculations [22] and magnetization measurements [23] , the magnetic moment in the D0 3 phase can be higher than the value for the B2 phase. Accordingly, short-range D0 3 -type ordering may cause a slight increase in the magnetic flux density in the matrix region, compared with the value expected for the ideal B2 phase. The impact of D0 3 -type short-range ordering needs to be studied further in the future. However, as the diffraction spots for the D0 3 phase are of diffuse scattering (distinct from the strong superlattice reflections due to B2-type ordering), we believe that the influence of D0 3 -type ordering is not significant in this specimen. The D0 3 -type structure order is invisible (that is, spots due to D0 3 -type ordering are absent) when the direction of the incident electrons is close to 〈001〉; refer to Fig. 1c . As the results in Figs 1b and 2 , 3 , 4 , 5 were obtained with electron incidence near (or exactly parallel to) 〈001〉, the observed APBs are related to the A2/B2 phase transformation; that is, the A2-type disordered APB layer separates the B2-type ordered regions, as illustrated in Fig. 1a . Measurements of magnetic flux density were also carried out at elevated temperatures, at 573 and 653 K, as shown in Fig. 5b,c . The values of B y measured for both the APB and matrix are plotted as a function of temperature in Fig. 5d . The error bar (±0.08 T) is mainly due to the uncertainty in measuring specimen thickness (see Supplementary Note 2 for details on the uncertainty). Although B y in the matrix was reduced to ~0.1 T or smaller at these elevated temperatures, the APB region continued to show significant magnetic flux density: 0.78 T at 573 K and 0.58 T at 653 K. The results reasonably explain the magnetic flux maps, such as those imaged in Fig. 4h,i , in which the ferromagnetic spin order persists in the narrow APB region. Because of time-consuming high-resolution electron holography experiments needed at elevated temperatures, we could determine the magnetic flux density of the APB only at three temperature points, 293, 573 and 653 K. For future examinations, it will be interesting to accurately determine the Curie temperature for both the APB and matrix regions based on the electron holography observations. These observations will also provide useful information for understanding the steps observed in the thermomagnetization curves in deformed Fe–Al alloys including disordered regions [33] , [34] , [35] . Nevertheless, the results in Fig. 4f–j and 5d explicitly indicate that the effective Curie temperature in the APB regions will be higher than that for the matrix. Our observations are unusual compared with those reported for other alloys in which atomic disordering in a thermal APB has only been believed to deteriorate ferromagnetic spin order [7] , [8] , [9] , [10] . Phenomenologically, the amplified magnetization can be explained by the framework concerned with nearest Fe–Fe pairs, which are responsible for the ferromagnetic spin order [17] , [20] , [22] , [23] , [24] . As factors affecting the number of nearest Fe–Fe pairs, we consider both atomic disordering and enrichment of the Fe content in the APB region. Based on EELS measurements, as shown in Fig. 3b , we assume the alloy composition in the APB region to be Fe 72 Al 28 ; that is, a slight increase in Fe content occurs compared with the value in the matrix, Fe 70 Al 30 . According to a report by Friák and Neugebauer [20] , binary Fe–Al alloys show a dramatic increase in magnetization (with increasing Fe content) in the Fe content range between 65 and 70%. In contrast, magnetization increases gradually over the Fe composition range higher than 70%. Ab initio calculations [20] indicated that the magnetic moment can be amplified by ~16% when the Fe content changes from 68.75 to 75%. It is unlikely to be that the amplified magnetization in APBs (amplified by 60% compared with the value in the matrix, at 293 K) can be explained only by the effect of compositional change. Calculations of site occupancy provide additional information for understanding this problem. For Fe–Al alloys showing a B2-type ordered cubic cell, which is composed of two simple cubic sublattices as shown in Fig. 1a , the number of nearest Fe–Fe pairs contained in 1-M unit of atoms ( N n ) is expressed by, where N 0 , z , P Fe I and P Fe II represent the Avogadro number, the coordination number, the Fe occupancy at corner sites (sublattice I) and the Fe occupancy at body-centred sites (sublattice II), respectively. For example, for the perfectly ordered state in Fe 70 Al 30 , P Fe I and P Fe II are 1.0 and 0.4, respectively (see left illustration in Fig. 1a ). The coordination number z =8 is used in the body-centred cell and the factor of 1/2 is included to avoid duplicate counting. For the Fe 70 Al 30 alloy, equation (4) yields N n =1.6 N 0 for the B2-ordered state, and N n =1.96 N 0 for the A2-disordered state ( P Fe I = P Fe II =0.7). This means that the atomic disordering increases the number of nearest Fe–Fe pairs by 22.5%. When we incorporate the Fe enrichment (~2%) into the calculations, the increase in the number of nearest Fe–Fe pairs becomes 29.6%, that is, comparison of the B2-ordered state in Fe 70 Al 30 and the A2-disordered state in Fe 72 Al 28 . The difference between these values (that is, 29.6–22.5%) can be a measure of the contribution from Fe enrichment on the increase in Fe–Fe nearest pairs; this corresponds to ~1/4 of the nearest pairs that are produced in the A2-disordered Fe 72 Al 28 . As far as these calculations are considered, we believe that the main cause of the amplified magnetization is breaking of the B2-type atomic order, which is responsible for ~3/4 of nearest pairs produced in the APB region. To explain the magnitude of the amplified magnetization (approximately 60% larger than the value of the matrix, observed at 293 K), we should consider additional factors indicated by researchers, such as the influence of the Fe–Fe distance on the magnetization [22] , [23] , [33] . In addition, determination of the degree of atomic order (for both matrix and APB regions) and/or deeper examination of Fe segregation are needed for a full understanding of this issue. These remain challenges for future studies. As briefly mentioned in the Introduction section, thermal APBs induce intriguing material functionalities such as pinning of magnetic domain walls [14] , unexpectedly large critical fields for magnetic saturation [13] and significant magnetoresistance [11] , [12] . All of these phenomena are related to the magnetic degradation that occurs in the APB regions showing atomic disordering. For example, the energy density of the magnetic domain wall can be minimized in an APB because of the depressed ferromagnetic exchange interaction [7] , [14] , [36] ; that is, the local energy change provides a pinning force against domain wall motion. In contrast, for ordered crystals used in spintronics (for example, spin-polarized Heusler alloys [15] ), depression of ferromagnetism may cause undesirable impedance of the spin-dependent electric current. In principle, it is difficult to remove thermal APBs from ordered crystals. Thus, tailoring the magnetism in the APB region is essential for further development of material functionalities in ordered alloys and compounds. Contrary to reports for many alloys and compounds (for example, Ni–Mn-based alloys [8] , [9] , Cu–Mn-based alloys [7] and inverse spinel-type magnetite [10] ), our observations have demonstrated that ferromagnetic spin order is developed in the APB region in Fe 70 Al 30 . Although the result may be predictable from previous theory [20] , [22] and experiments [16] , [17] , [18] , [19] , [23] , [24] , [33] , [34] , [35] , which were used to intensively study the relationship between atomic disorder and magnetization in Fe–Al alloys, our study revealed that this relationship can be achieved even in nanometre-scale, thermally induced APBs. The observations imply an important role of atomic disordering of Fe within the body-centred cubic lattice on the tuning of ferromagnetism in the APB region. For further examinations relevant to materials design and/or tailoring of APB-induced phenomena, electron holography can be applied to other Fe-based bcc alloys. We also emphasize that the advanced techniques of electron holography used in this work achieved pin-point magnetization analysis from the nanometre-sized interface region. The methods can be widely applied to leading problems in spintronics, physics, chemistry and materials science. Specimen preparation To study the magnetization in the narrow APB region, we chose the alloy composition Fe 70 Al 30 , which provided favourable conditions for electron microscopy experiments for the following reasons. For alloys with an Fe content higher than 70%, it was difficult to suppress the development of long-range D0 3 -type ordering, that is, the specimens showed complex microstructures with APBs related to the D0 3 /B2 phase transformation, in addition to APBs related to the B2/A2 phase transformation. For alloys with an Fe content <70%, spontaneous magnetization is reduced, making magnetic flux density measurement by electron holography difficult. Fe 70 Al 30 alloy is ideal for avoiding these problems. An ingot of Fe 70 A 30 alloy was heat-treated at 1,473 K for 12 h, followed by quenching in ice water. Thin-foil specimens for TEM studies were prepared by electrochemical polishing. The specimens definitively showed B2-type ordering, as demonstrated by the superlattice reflections indicated by red circles in the electron diffraction patterns ( Fig. 1c,d ). The size of the antiphase domains was on the order of 100 nm. Cross-sectional TEM observations evaluated the specimen thickness at the region of interest (that is, the position at which the magnetic flux density data shown in Fig. 5 were determined) to be ~79 nm. There was no preferential etching at APB positions (that is, steep change in thickness at the APB positions), as mentioned in Supplementary Note 1 . Electron microscopy observations High-angle annular dark-field scanning TEM and EELS observations were carried out using a 200-kV transmission electron microscope (JEM-ARM200F, JEOL). Electron holography experiments, Lorentz microscopy and bright-field/dark-field imaging were conducted using a 300-kV electron microscope (HF-3300S, Hitachi). When the electron holograms and Lorentz microscopy images were collected, the specimen was subjected to a negligible magnetic field (of the same order as the geomagnetic field) due to the shielding design of the microscope. To examine the magnetization distribution in the narrow APB region, we employed split-illumination electron holography [28] . This method enabled illumination of the APB area with sufficiently high beam intensity, which improved the signal-to-noise ratio in the electron holograms. For the view field shown in Fig. 4 , Lorentz microscopy visualized the portions showing amplified magnetization along the APBs, which were imaged as paired bright and dark lines due to magnetic deflection of incident electrons by the Lorentz force. The images were recorded using a charge-coupled device camera (USC 4000, Gatan). To suppress undesired diffraction contrast, the specimen was slightly inclined when the electron holograms were acquired. How to cite this article: Murakami, Y. et al. Magnetization amplified by structural disorder within nanometre-scale interface region. Nat. Commun. 5:4133 doi: 10.1038/ncomms5133 (2014).